High-temperature electromagnons in the magnetically induced multiferroic cupric oxide driven by intersublattice exchange Magnetically induced ferroelectric multiferroics present an exciting new paradigm in the design of multifunctional materials, by intimately coupling magnetic and polar order. Magnetoelectricity creates a novel quasiparticle excitation—the electromagnon—at terahertz frequencies, with spectral signatures that unveil important spin interactions. To date, electromagnons have been discovered at low temperature (<70 K) and predominantly in rare-earth compounds such as R MnO 3 . Here we demonstrate using terahertz time-domain spectroscopy that intersublattice exchange in the improper multiferroic cupric oxide (CuO) creates electromagnons at substantially elevated temperatures (213–230 K). Dynamic magnetoelectric coupling can therefore be achieved in materials, such as CuO, that exhibit minimal static cross-coupling. The electromagnon strength and energy track the static polarization, highlighting the importance of the underlying cycloidal spin structure. Polarized neutron scattering and terahertz spectroscopy identify a magnon in the antiferromagnetic ground state, with a temperature dependence that suggests a significant role for biquadratic exchange. Multiferroic materials exhibit multiple ferroic orders, such as ferromagnetism and ferroelectricity, although materials that are antiferromagnetic (AFM) and ferroelectric are also widely termed multiferroic [1] , [2] , [3] . In magnetoelectric multiferroics these properties are intimately coupled, allowing the electrical switching of magnetization or vice versa. Strong magnetoelectric coupling can be achieved in materials with spin cycloid structures that induce electrical polarization [4] , [5] . Deepening our fundamental understanding of the static and dynamic magnetoelectric effects is vital to obtain the enhanced ferroic properties and coupling necessary for room temperature multiferroic devices. The static polarization of induced multiferroics such as R MnO 3 ( R : rare earths) can be understood as arising from the spin current or inverse Dzyaloshinskii–Moriya interaction [6] , whereby spin-orbit coupling produces a polarization proportional to the cross-product of adjacent spins ( S i × S j ). In contrast, the dynamic response under oscillating fields can elucidate other significant interactions. Magnetoelectric coupling creates a new quasiparticle excitation—the electromagnon—at terahertz (THz) frequencies [7] , [8] , [9] , [10] , [11] , [12] , [13] . Electromagnons have been discovered in rare-earth-doped compounds such as R MnO 3 and R Mn 2 O 5 at low temperature (<70 K), and are thought to result from modifications of the Heisenberg exchange interaction [14] , [15] , which has a S i · S j term in the spin Hamiltonian. Single-ion anisotropy (SIA) and biquadratic exchange (BE) are required to capture fully the spectral features of electromagnons in the THz range [16] . Novel device concepts that utilize electromagnons or electrically tuned magnons [17] , [18] are contributing to the emerging field of magnonics, which aim to use spin waves in data processing and communications [19] . Exceptionally among the 3 d -transition metal monoxides, cupric oxide (CuO) is a multiferroic with magnetically induced ferroelectricity [20] . Neutron diffraction studies have clarified the magnetic phases of CuO [21] , [22] . At low temperatures there is a commensurate, collinear antiferromagnetic phase (AF1) with two Cu 2+ sublattices, on which spins are oriented parallel or anti-parallel to [010], as pictured in Fig. 1 . The nearest neighbour exchange interactions responsible for the AF1 ground state are as follows (in the numbering convention of ref. 23 ). The strongest exchange, J 1 , is AFM and occurs along spin chains in the direction ( Fig. 1 ). Weaker ferromagnetic (FM) coupling exists between chains on the same sublattice in the [101] and [010] directions, given by J 2 and J 7, respectively [24] . Between 213 and 230 K (AF2 phase) the spins on one sub-lattice rotate into the ac -plane [21] , [22] , [25] , as pictured in Fig. 1b , and an incommensurate spin spiral structure is formed with magnetic modulation vector Q =(0.006, 0, 0.017). The incommensurate structure is essentially a cycloid, with a small proper screw component, and is visualized along Q in Fig. 1c . This phase exhibits a static electric polarization P b ~100 μC m −2 along b [20] , [26] , [27] , the origin of which has been discussed in the context of weakly frustrated intersublattice spin interactions [23] , magnetic degeneracy and the spin-orbit interaction [28] and cross-coupled AFM order parameters [29] . While CuO exhibits ferroelectric hysteresis loops [20] and chiral magnetic domains that can be switched electrically [27] , no substantial uniform static magnetoelectric coupling has been found in polycrystalline CuO up to 7 T [26] , and the AF2 phase appears to be stable to at least 16 T [30] . Intriguingly, hydrostatic pressure has been suggested to broaden the temperature width of the multiferroic phase past room temperature [31] . 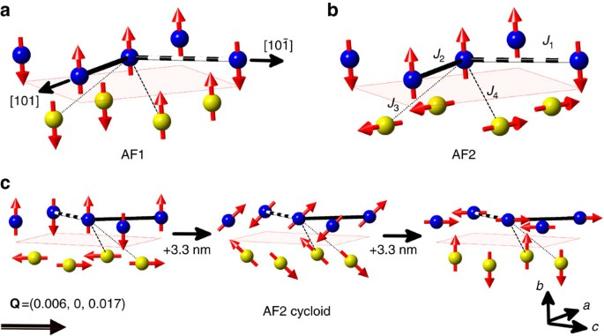Figure 1: Local spin structure in CuO. (a) In the AF1 phase, below 213 K, spins lay in the ±b-direction. (b) In the AF2 phase (213–230 K) spins on one Cu sublattice re-orient into theac-plane. The two different Cu sublattices are shown in blue and yellow, while the shaded area indicates theac-plane. The exchange constantJ1in thedirection creates antiferromagnetic order, while in the [101] directionJ2is ferromagnetic.J3andJ4describe the exchange interaction between sublattices. (c) Incommensurate AF2 spin structure for three unit cells along the magnetic modulation vectorQ=(0.006, 0, 0.017). Spins rotate in the plane containingbandε=0.506a*+1.517c* (refs21,22). Lattice vectorsa,bandcjust refer to subplot (c). Figure 1: Local spin structure in CuO. ( a ) In the AF1 phase, below 213 K, spins lay in the ± b -direction. ( b ) In the AF2 phase (213–230 K) spins on one Cu sublattice re-orient into the ac -plane. The two different Cu sublattices are shown in blue and yellow, while the shaded area indicates the ac -plane. The exchange constant J 1 in the direction creates antiferromagnetic order, while in the [101] direction J 2 is ferromagnetic. J 3 and J 4 describe the exchange interaction between sublattices. ( c ) Incommensurate AF2 spin structure for three unit cells along the magnetic modulation vector Q =(0.006, 0, 0.017). Spins rotate in the plane containing b and ε =0.506 a *+1.517 c * (refs 21 , 22 ). Lattice vectors a , b and c just refer to subplot ( c ). Full size image Here we report that CuO exhibits a sizeable dynamic magnetoelectric response. THz time-domain spectroscopy (THz-TDS) uncovered an electromagnon excitation linked to the multiferroic phase, at the highest temperature reported to date for magnetically induced ferroelectricity. Insights into the relevant microscopic interactions are gained by examining THz spectra in both the non-polar AFM state and the polar multiferroic phase, and emphasize the importance of BE and intersublattice spin interactions in CuO. Room temperature THz dielectric tensor Monoclinic CuO is a biaxially birefringent material, with a dielectric tensor ε ij that consists of a scalar term ε y = ε b along [010] and a matrix term in the ac -plane when expressed in a Cartesian co-ordinate system [32] with x ‖ a , y ‖ b , z ‖ c *. A combination of transmission and reflection geometry THz-TDS was used to determine the complex refractive index at room temperature in the paramagnetic (PM) insulating phase ( μ ij =1) over the energy range 0.8–23 meV (0.2–5.5 THz), as reported in Fig. 2 . A variety of crystal orientations were examined. The birefringence of CuO is largest between [010] and the ac -plane, and can be witnessed directly in the time domain in Fig. 2a at various sample azimuthal angles ϕ , where ϕ =0 corresponds to [101]. The real part of the refractive index is reported in Fig. 2b and the absorption in Fig. 2c . The data on the left (right) were taken in transmission (reflection), allowing the characterisation of the lowest transverse optical phonon modes for E [101] and E [010] . The mode is at 21.1 meV (5.1 THz), and is driven by E [010] , while an electric field in the ac -plane excites the mode at 19.0 meV (4.6 THz) [32] , [33] . Here the superscripts label the normal modes. 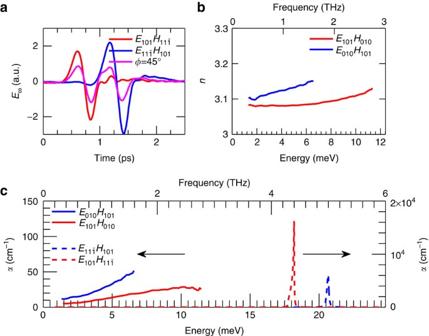Figure 2: THz dielectric response of CuO at room temperature. (a) The transmitted THz electric field in the time domain shows the sample’s birefringence: whenEωis aligned with one of the optical axes a single cycle pulse is visible, whereas two pulses arise whenEωhas equal components along each of fast and slow axes (ϕ=45°). (b) Real part of the refractive index shown forEωin theac-plane (red) and along thebaxis (blue). (c) Complementary absorption data from transmission (left) and reflection (right) measurements. Figure 2: THz dielectric response of CuO at room temperature. ( a ) The transmitted THz electric field in the time domain shows the sample’s birefringence: when E ω is aligned with one of the optical axes a single cycle pulse is visible, whereas two pulses arise when E ω has equal components along each of fast and slow axes ( ϕ =45°). ( b ) Real part of the refractive index shown for E ω in the ac -plane (red) and along the b axis (blue). ( c ) Complementary absorption data from transmission (left) and reflection (right) measurements. Full size image The [101], and [010] directions are optical axes [32] , and at intermediate ϕ time-domain components are visible for each axis ( Fig. 2a ). A misorientation of the sample of ϕ ~10° can create spectral artefacts in the absorption coefficient α when calculated using a vacuum reference. In the subsequent analysis, we therefore report the absorption change Δ α relative to the AF1 phase or the PM phase. This also alleviates the influence of absorption created by the mode at 51.3 meV (12.4 THz) [32] , which dominates the absorption below 12 meV for E [010] owing to its substantial linewidth (maximum 7.7 meV or 1.9 THz), as demonstrated in Supplementary Fig. 1 ; Supplementary Note 1 . Dynamic magnetoelectric response To examine the THz response of CuO in the non-polar AF1 and polar AF2 phases the relative absorption Δ α ( T )= α ( T )− α ( T 0 ) is shown for a variety of E ω and H ω orientations in Fig. 3 . The absorption relative to T 0 =200 K is shown in Fig. 3a for E [101] with either H [010] or . Representative temperatures T chosen were 212 K (AF1 phase), 216 K (AF2 phase) and 246 K, in the PM phase. A significant absorption for E [101] (Δ α =4–10 cm −1 ) is present in the multiferroic AF2 phase, centered at 2.9 meV (0.7 THz), with linewidth ~2 meV (0.5 THz), and which is not present in the AF1 and PM phases. This mode is present irrespective of the direction of the magnetic field of the THz radiation, H [010] or . In contrast, no such resonance is observed when the electric field is oriented along [010] or ( Fig. 3b ). Therefore this mode is an electric-dipole active magnon—an electromagnon—driven by E [101] . The maximum value of Δ α varies somewhat between samples, suggesting a possible influence of crystal alignment or of sampling multiple domains. For reference, the absolute absorption coefficient α is reported in Supplementary Fig. 2a . 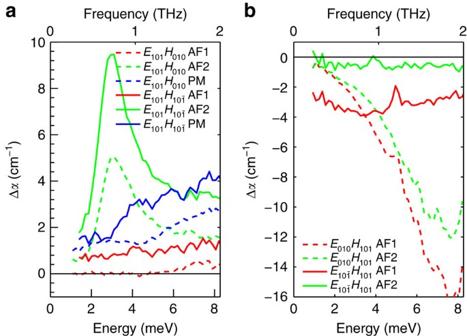Figure 3: Relative THz absorption spectra of CuO in each magnetic phase. (a) Spectra forEω‖(101) withHωalong(solid lines) and (010) (dashed lines) show a strong absorption at 2.9 meV (0.7 THz) in the AF2 phase (216 K) only. (b) Complementary spectra withHω‖(101) andEωalong(solid lines) and (010) (dashed lines) show a weaker absorption at 5.0 meV (1.2 THz) in the AF1 phase (200 K) and at 4 meV (0.97 THz) in the AF2 phase. Figure 3: Relative THz absorption spectra of CuO in each magnetic phase. ( a ) Spectra for E ω ‖ (101) with H ω along (solid lines) and (010) (dashed lines) show a strong absorption at 2.9 meV (0.7 THz) in the AF2 phase (216 K) only. ( b ) Complementary spectra with H ω ‖ (101) and E ω along (solid lines) and (010) (dashed lines) show a weaker absorption at 5.0 meV (1.2 THz) in the AF1 phase (200 K) and at 4 meV (0.97 THz) in the AF2 phase. Full size image The relative absorption coefficient for H [101] (with E [010] and ) are presented in Fig. 3b , where a reference at T 0 =246 K was used for all data. This highlights a weak, narrow absorption feature in the AF1 phase more clearly. At T =200 K an enhanced absorption at 5.0 meV (1.2 THz) is clearly visible for , while for E [010] this resonance appears as a shoulder superimposed on a decrease in Δ α created by the broad phonon mode [32] . The resonance loses oscillator strength rapidly at the AF1/AF2 phase boundary, where spins on one sub-lattice rotate to lie in the ac -plane, and is weakly visible at 4 meV (0.97 THz) at 216 K (green, solid line). It can be identified as a pure spin-wave resonance (a magnon) with minimal spin-lattice coupling because: (i) it is present in the AF1 phase, (ii) it is present for H [101] regardless of the direction of E and (iii) it has weaker spectral weight and sharper linewidth (<0.08 meV at 10 K, ~0.4 meV at 216 K) in comparison with the electromagnon (~1.2 meV at 213 K). Magnon resonances are typically observed at THz frequencies in oxides and fluorides with AFM nearest neighbour coupling, while for materials with FM coupling they lie in the GHz range [34] , [35] . CuO exhibits both AFM ( J 1 along ) and FM ( J 2 along [101] and J 7 along [010]) nearest neighbour coupling in its low-temperature phase. Electromagnon In order to elucidate the nature of the electromagnon excitation ( E [101] ), we present in Fig. 4a Δ α up to 10.3 meV (2.5 THz) in the temperature range 210–235 K. The electromagnon appears rapidly (within 0.3 K) at the AF1/AF2 phase transition, and consists of a strong peak at 3 meV and a weaker shoulder from 4–6 meV. The static polarization P [010] was obtained from pyroelectric current measurements in the [010] direction (sample with [101] and crystal axes in the plane) [27] , and is shown in Fig. 4b . The excitation energy ( Fig. 4c ) and absorption strength ( Fig. 4d ) of the electromagnon closely track P [010] , supporting this mode’s assignment as an electromagnon, and suggesting that it is intimately linked to the cycloidal spin structure of the AF2 phase. 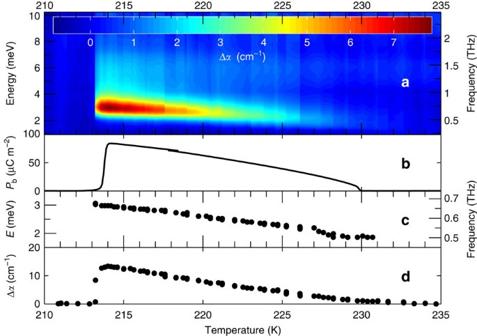Figure 4: Temperature dependence of THz absorption and static polarization. (a) The evolution of the terahertz absorption coefficient Δαwith temperature. The sharp onset of the electromagnon mode at the AF1/AF2 phase boundary is followed by a gradual decrease in mode frequency and strength to the AF2/PM boundary. (b) The static electric polarizationPb(obtained from the pyroelectric current), (c) electromagnon energy and (d) absorption strength exhibit the same temperature dependence. The data in (b) are reproduced with permission from ref.27. Figure 4: Temperature dependence of THz absorption and static polarization. ( a ) The evolution of the terahertz absorption coefficient Δ α with temperature. The sharp onset of the electromagnon mode at the AF1/AF2 phase boundary is followed by a gradual decrease in mode frequency and strength to the AF2/PM boundary. ( b ) The static electric polarization P b (obtained from the pyroelectric current), ( c ) electromagnon energy and ( d ) absorption strength exhibit the same temperature dependence. The data in ( b ) are reproduced with permission from ref. 27 . Full size image In Supplementary Fig. 2b ; Supplementary Note 2 , a Drude–Lorentz oscillator fit to the electromagnon absorption is reported. The strength Δ ε =0.075 of this electromagnon is weaker than the E ω ‖ a electromagnons reported in TbMnO 3 (Δ ε =2), thought to arise from the Heisenberg exchange mechanism [14] , and comparable to that assigned to an eigenmode of the spin cycloid (Δ ε =0.05) [12] . Previously, the application of an optical sum rule has shown that electromagnons in R Mn 2 O 5 account for step-like changes in the static dielectric constant [9] . In Supplementary Fig. 3 the change in dielectric constant is reported at 0.2 THz as obtained directly from THz-TDS, along with that obtained from the sum rule analysis described in Supplementary Note 3 . A significant step-like increase in dielectric constant along [101] at 213 K can be observed to result from electromagnons. Dielectric measurements between 100 Hz and 100 kHz have previously been reported for the b axis only [20] , and show anomalies at the AF1/AF2 and AF2/PM transition temperatures. The static polarization of rare-earth perovskite manganites (for example, R MnO 3 , where R =Tb, Dy) can be explained by the inverse Dzyaloshinskii–Moriya interaction [11] , [36] , in which a spin cycloid breaks inversion symmetry. In contrast, the dynamic polarization at THz frequencies is dominated by electromagnons [11] , [13] , [14] , [37] created by spin-lattice coupling, with the following term in the Hamiltonian: As CuO is an improper multiferroic analogous to R MnO 3 and R Mn 2 O 5 , with comparable static polarization and cycloidal spin structure [20] , electromagnon models [15] , [16] developed for these compounds may be expected to apply. An electric field displaces ions a distance u k along direction k , altering the bond angles along Cu–O–Cu superexchange pathways and thus J n . The local magnetic field experienced by each spin S i is . The dynamical motion of spins can then be derived from the Landau–Lifshitz–Gilbert equation [15] , [16] , yielding if damping is ignored. Electric fields can thus drive spin oscillations only if S i and S j are not parallel. For CuO, only the intersublattice superexchange terms J 3 and J 4 couple non-parallel spins, as depicted in Fig. 1b . The electromagnon is only excited by E [101] , that is, along the FM CuO chains, altering both intersublattice exchange pathways. The contribution of additional interactions to the spin Hamiltonian can be understood by examining electromagnon spectra. Two or more absorption peaks are witnessed for R MnO 3 [11] , [13] . The peak at higher energy can be understood by models including only Equation 1 [11] , [14] , while the addition of SIA and BE terms is necessary to model the lower energy electromagnon [16] . In comparison, the electromagnon spectra in Figs 3a and 4a exhibit more significant spectral weight at lower frequencies, suggesting that SIA or BE plays a significant role in the multiferroic phase of CuO. The experimental Δ α ( T =216 K) can be fit using two Drude–Lorentz oscillators, as described in Supplementary Fig. 2b . Magnon To examine the AF1 ground state of CuO, we investigated the temperature dependence of the magnon ( H [101] ) resonance, which redshifts with increasing temperature, as indicated by the crosses in Fig. 5a . Also shown is the electromagnon frequency (squares), which is reduced for a mixed spin-lattice mode with respect to the pure magnon frequency [38] . We constructed a phenomenological spin model for the magnon using a linear and biquadratic superexchange model [39] that was utilized recently to model the temperature dependence of the THz AFM resonance in MnO [40] . Details of this model are given in the Supplementary Note 4 . We assume that the exchange energy per Cu 2+ ion is given by U =− J σ 2 S 2 − j σ 4 S 4 , where σ is the reduced sub-lattice magnetization, and J and j describe the total linear and quadratic nearest neighbour exchange interactions [39] . 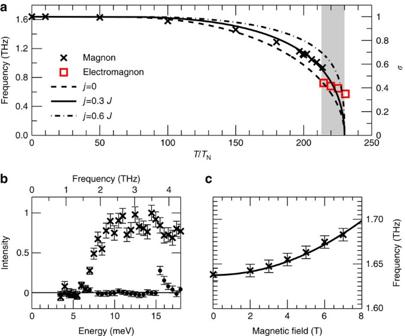Figure 5: Temperature and magnetic-field dependence of the magnon resonance. (a) The temperature dependence of theH[101]magnon mode (crosses) tracks the sub-lattice magnetizationσ(lines) calculated from a phenomenological model described in the text. Good agreement is found for a biquadratic exchange ratio ofj/J=0.3 (solid line), rather than withj=0 (dashed) orj/J=0.6 (dash-dotted line). (b) Polarized inelastic neutron-scattering spectra at 10 K show the separated transverse magnetic (crosses) and nuclear (points)-scattering signal at Q=(−0.5, 0, −1.5). The error bars are derived from the square root of the raw detector counts. A gap in the magnon spectrum at 7.75 meV correlates with the magnon resonance frequency in subplot (a). (c) The magnon frequency at 10 K (points) increases quadratically (line) with a static magnetic field along [010]. Errors are calculated from the residuals of fits to magnon oscillations in the time domain. Figure 5: Temperature and magnetic-field dependence of the magnon resonance. ( a ) The temperature dependence of the H [101] magnon mode (crosses) tracks the sub-lattice magnetization σ (lines) calculated from a phenomenological model described in the text. Good agreement is found for a biquadratic exchange ratio of j / J =0.3 (solid line), rather than with j =0 (dashed) or j / J =0.6 (dash-dotted line). ( b ) Polarized inelastic neutron-scattering spectra at 10 K show the separated transverse magnetic (crosses) and nuclear (points)-scattering signal at Q=(−0.5, 0, −1.5). The error bars are derived from the square root of the raw detector counts. A gap in the magnon spectrum at 7.75 meV correlates with the magnon resonance frequency in subplot ( a ). ( c ) The magnon frequency at 10 K (points) increases quadratically (line) with a static magnetic field along [010]. Errors are calculated from the residuals of fits to magnon oscillations in the time domain. Full size image The temperature dependence of the magnon frequency, assumed to be proportional to the sublattice magnetization [34] , was then determined from A ratio j / J =0.3 produced an excellent accord with experiment, as evidenced by the solid line in Fig. 5a . The cases with zero ( j =0, dashed line) and stronger BE ( j / J =0.6, dash-dotted line) resulted in poorer agreement. Previous studies have suggested that BE may play an important role in determining the spin structure of CuO. By constructing a mean-field theory for weakly coupled AFM spin chains, Yablonskii [25] showed that the inclusion of BE can stabilize the commensurate state at low temperature, and the incommensurate phase at an elevated temperature [41] . Recent variational calculations combined with Monte Carlo simulations [42] have also highlighted BE interactions as important in stabilizing incommensurate magnetic states at finite temperature, as in CuO. The temperature dependence of the magnon frequency therefore provides experimental evidence consistent with BE, although alternative microscopic mechanisms may result in the same phenomenology. Note that the fit to the reduced temperature depends on j / J rather than J . Neutron scattering has determined J 1 to be between −75 and −80 meV, with J 2 =5 and J 7 =3 meV [24] , [43] . Other measurements include | J 1 |=77 meV from susceptibility [44] , and | J 1 |=100 meV from mid-infrared conductivity [45] and Raman spectra [46] . Recent DFT calculations have yielded values for J 1 ranging from −51 to −127 meV [23] , [28] . Polarized neutron scattering was utilized to probe further the AF1 phase. Polarization analysis [47] was used to separate the magnetic and nuclear scattering. In Fig. 5b magnetic (crosses) and nuclear (points)-scattering spectra are reported for the AFM wavevector Q=(−0.5,0,−1.5) at T =10 K. The magnetic scattering corresponds to spin fluctuations perpendicular to Q in the ac -plane. A sharp gap for in-plane magnetic fluctuations at 7 meV correlates well with the magnon resonance observed with THz-TDS at 6.8 meV (1.64 THz, Fig. 5a ), demonstrating that the magnon is linked to ac -plane spin fluctuations. There is no nuclear scattering until a low-energy phonon mode at 15.5 meV, which derives from an acoustic branch [48] . The magnetic field dependence of the magnon resonance was investigated by applying a static field parallel to the b axis of an ac -plane oriented sample, and probing H [101] with THz-TDS. As illustrated in Fig. 5c , the magnon frequency increases quadratically with field in the range 0–7 T. This is consistent with high-frequency electron spin resonance (ESR) measurements in fields up to 40 T [49] . The ESR data show additional modes around 300 GHz associated with the collinear phase and the spin-flop transition at 10.2 T [49] , [50] . In summary, the dynamic magnetoelectric response of the multiferroic CuO was investigated. An electromagnon excitation was discovered in the multiferroic phase (213–230 K), and was attributed to spin-lattice coupling between different Cu spin sublattices. The electromagnon spectrum, and temperature dependence of the magnon frequency, indicate that CuO exhibits a sizable magnetic anisotropy. The observation of electromagnons in an improper multiferroic at close to room temperature may create exciting new prospects for magnonic devices operating at THz frequencies. In the commensurate magnetic phase a magnon resonance observed via THz spectroscopy correlates with a gap in the in-plane magnetic-scattering component from inelastic neutron scattering. Sample growth and characterization Single crystals of CuO (monoclinic, space group C 2/c [51] ) were grown by the optical float zone method [52] . The boule was oriented by X-ray Laue diffraction and flat, plate-like samples were cut and polished with the following in-plane crystallographic directions: (101) and (010); (101) and ; (101) and . High resolution ω −2 θ X-ray scans confirmed that samples were single crystals. Superconducting quantum interference device measurements of the magnetic susceptibility were in agreement with results in the literature [20] , [27] . THz-TDS THz-TDS [53] was used to probe the dynamic magnetoelectric response in the energy range 0.8 – 12.4 meV (0.2–3 THz), for sample temperatures from 2 to 300 K and magnetic fields to 7 T. THz-TDS directly determines the amplitude of the electric field E ω after interaction with the sample, providing knowledge of the complex refractive index . Using linearly polarized THz radiation and an appropriate combination of sample orientations [54] the dielectric and magnetic contributions to ñ were determined. Polarized neutron scattering The polarized neutron-scattering experiments were performed on the IN20 spectrometer, at the Institut Laue-Langevin in Grenoble, France. Polarization analysis [47] was used to separate the magnetic and nuclear-scattering contributions. A single crystal, of mass 6.7 g and a crystal mosaic <2° was aligned with ( h , 0, l ) as the scattering plane. The monochromator and analyser used were both polarizing Heusler (111) crystals and the measurements were taken at a fixed final wavevector of k f =2.662 Å. How to cite this article: Jones, S. P. P. et al . High-temperature electromagnons in the magnetically induced multiferroic cupric oxide driven by intersublattice exchange. Nat. Commun. 5:3787 doi: 10.1038/ncomms4787 (2014).